MS-GF+ makes progress towards a universal database search tool for proteomics Mass spectrometry (MS) instruments and experimental protocols are rapidly advancing, but the software tools to analyse tandem mass spectra are lagging behind. We present a database search tool MS-GF+ that is sensitive (it identifies more peptides than most other database search tools) and universal (it works well for diverse types of spectra, different configurations of MS instruments and different experimental protocols). We benchmark MS-GF+ using diverse spectral data sets: (i) spectra of varying fragmentation methods; (ii) spectra of multiple enzyme digests; (iii) spectra of phosphorylated peptides; and (iv) spectra of peptides with unusual fragmentation propensities produced by a novel alpha-lytic protease. For all these data sets, MS-GF+ significantly increases the number of identified peptides compared with commonly used methods for peptide identifications. We emphasize that although MS-GF+ is not specifically designed for any particular experimental set-up, it improves on the performance of tools specifically designed for these applications (for example, specialized tools for phosphoproteomics). Mass spectrometry (MS) instruments and experimental protocols have greatly advanced over the last decade. New fragmentation technologies have emerged and high-precision mass spectrometers like Orbitrap have become widely available. Although trypsin remains a dominant protease in proteomics studies, digesting proteins with diverse proteases is becoming popular [1] . Empowered by these changes, MS researchers now have diverse choices with respect to the questions: ‘what fragmentation method to use?’, ‘how accurate should be the measurements of the mass-to-charge ( m/z ) ratios?’, ‘what proteases to use?’ and ‘what post-translational modification (PTM) to focus on (for example, phosphorylation)?’. Depending on these choices, the resulting tandem mass (MS/MS) spectra vary in fragmentation propensities and precision. Therefore, unlike in the past when low-precision collision-induced dissociation (CID) spectra of tryptic peptides dominated the field, spectral data sets generated today are very diverse. Unfortunately, the popular MS/MS database search tools such as SEQUEST [2] and Mascot [3] have not kept pace with the increased diversity of the data. Although several new MS/MS database search engines were recently developed, including Andromeda [4] , Morpheus [5] , and MS Amanda [6] , they have resulted in only minor improvements as compared with SEQUEST and Mascot. Many efforts have been invested into making existing MS/MS search tools compatible with new types of data. For example, several pre- or post-processing strategies have been proposed [7] , [8] , resulting in small improvement in the performance of database search tools. To further boost the performance, MS/MS database search tools are combined with statistical modelling tools such as PeptideProphet [9] , Percolator [10] and IDPicker [11] . These tools do not find new peptide–spectrum matches (PSMs), but rather re-score PSMs reported by a database search tool using more complex scoring and output high-scoring PSMs. Although they often improve the performance of a database search tool, their performance is negatively affected when the database search tool fails to find correct PSMs [12] . Another downside of the pre- or post-processing strategies and statistical modelling tools is that, as they are often not integrated into database search tools, using them complicates the analysis of MS/MS spectra. Moreover, as different laboratories employ different combinations of tools (see Fig. 1 ), even for the same data, capabilities of analysing the data vary widely and results obtained in one laboratory are often difficult to reproduce in another laboratory [13] . 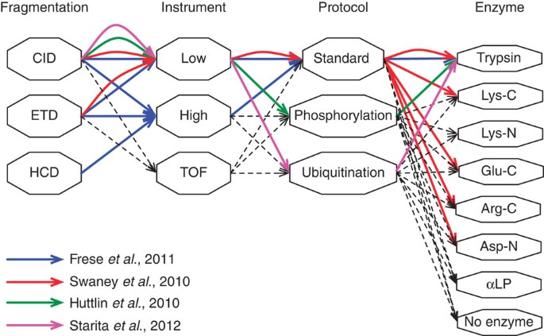Figure 1: Various spectral types. Spectral types are represented as paths in the graph representing possible choices of the fragment method (Fragmentation), the instrument measuring product ionm/z(Instrument), the protocol used to prepare a sample (Protocol) and the enzyme used to digest proteins (Enzyme). ‘Low’ in Instrument indicates low-resolution instruments (for example, linear ion trap), ‘High’ indicates high-resolution instruments (for example, Orbitrap) and ‘TOF’ indicates time-of-flight instruments. ‘Phosphorylation’ and ‘Ubiquitination’ in Protocol indicate that spectra are generated from phosphopeptides and ubiquitinated peptides, respectively. A path in the graph represents a spectral type. For example, the green path (CID, Low, Phosphorylation, Trypsin) represents low-precision CID spectra of trypsin digests generated from a sample enriched for phosphopeptides. The blue, red, green and magenta paths represent spectral types of the data sets used in recent studies by Freseet al.20, Swaneyet al.1, Huttlinet al.21and Staritaet al.22, respectively. Different combinations of analysis tools were used for different studies. Freseet al.used an in-house tool for peak filtering, de-isotoping, and charge deconvolution, Mascot for database search, Percolator for re-scoring, and RockerBox58for peptide-level FDR control. Swaneyet al.1used an in-house tool for peak filtering, OMSSA27for database search and an in-house tool for both peptide- and protein-level FDR control. Huttlinet al.21used an in-house tool for re-calibrating peak masses, SEQUEST for database search, an in-house tool for re-scoring and peptide- and protein-level FDR control. Staritaet al.22used the Trans-Proteomics Pipeline45along with SEQUEST for database search. The same data sets were analysed by MS-GF+ without using any additional tool with scoring parameters trained separately for different spectral types. Figure 1: Various spectral types. Spectral types are represented as paths in the graph representing possible choices of the fragment method (Fragmentation), the instrument measuring product ion m/z (Instrument), the protocol used to prepare a sample (Protocol) and the enzyme used to digest proteins (Enzyme). ‘Low’ in Instrument indicates low-resolution instruments (for example, linear ion trap), ‘High’ indicates high-resolution instruments (for example, Orbitrap) and ‘TOF’ indicates time-of-flight instruments. ‘Phosphorylation’ and ‘Ubiquitination’ in Protocol indicate that spectra are generated from phosphopeptides and ubiquitinated peptides, respectively. A path in the graph represents a spectral type. For example, the green path (CID, Low, Phosphorylation, Trypsin) represents low-precision CID spectra of trypsin digests generated from a sample enriched for phosphopeptides. The blue, red, green and magenta paths represent spectral types of the data sets used in recent studies by Frese et al. [20] , Swaney et al. [1] , Huttlin et al. [21] and Starita et al. [22] , respectively. Different combinations of analysis tools were used for different studies. Frese et al. used an in-house tool for peak filtering, de-isotoping, and charge deconvolution, Mascot for database search, Percolator for re-scoring, and RockerBox [58] for peptide-level FDR control. Swaney et al. [1] used an in-house tool for peak filtering, OMSSA [27] for database search and an in-house tool for both peptide- and protein-level FDR control. Huttlin et al. [21] used an in-house tool for re-calibrating peak masses, SEQUEST for database search, an in-house tool for re-scoring and peptide- and protein-level FDR control. Starita et al. [22] used the Trans-Proteomics Pipeline [45] along with SEQUEST for database search. The same data sets were analysed by MS-GF+ without using any additional tool with scoring parameters trained separately for different spectral types. Full size image In a recent review, Noble and MacCoss [14] pointed out that ‘the field (of MS) is still missing a generic analysis platform that can be adapted automatically and in a principled manner, to handle spectra produced by any given fragmentation protocol’. Our MS-GF+ is a step towards achieving this goal, representing a universal database search tool that performs well for diverse types of spectral data sets. MS-GF+ works well (that is, identifies more peptides than other MS/MS tools that we tested) for spectra generated using diverse configurations of MS instruments and experimental protocols. However, the main contribution of this study is not the increase in the number of identifications for dozens of various fragmentation methods and experimental protocols but rather the fact that it represents the first truly universal MS/MS database search tool. We emphasize that MS-GF+ is not customized for specific spectral data sets but rather uses a robust probabilistic model that works well across all data sets. MS-GF+ is universal because it automatically derives scoring parameters from thousands of PSMs without prior knowledge of the type of the spectra [12] . We represent various types of spectra as a graph where paths represent spectral types ( Fig. 1 ). For each spectral type, MS-GF+ learns scoring parameters separately and scores a PSM using a different set of scoring parameters depending on the spectral type. MS-GF+ can train scoring parameters for any spectral type (including spectral types not specified in Fig. 1 ) or use pre-trained scoring parameters. It takes over the authority to train scoring parameters to the users and makes the training easy. The key advantage of MS-GF+ over existing approaches is its ability to compute rigorous E -values (using the generating function approach [15] ) and thus to boost the number of peptide identifications. Although the generating function approach from ref. 15 worked well in a variety of studies [16] , [17] , [18] , [19] , the question of applying it to modified peptides and to high-precision MS/MS spectra remains open. In this study we address these issues, thus making the generating function approach applicable to all types of spectra. We demonstrate the performance of MS-GF+ using various previously studied data sets [1] , [20] , [21] , [22] , [23] : spectra of tryptic peptides generated using CID, higher-energy collisional dissociation (HCD) and electron transfer dissociation (ETD) in combination with either linear ion trap or Orbitrap readout, spectra of multiple enzyme digests, spectra of phosphopeptides and spectra or a novel protease alpha-lytic protease (αLP). For all these data sets, we show that MS-GF+ outperforms popular tools for peptide identification such as Mascot+Percolator. MS-GF+ scoring Database search tools use a scoring function Score( P , S ) to evaluate a PSM of a peptide P and a spectrum S , and further compute statistical significance of the resulting PSMs. In this study, we use E -values to evaluate statistical significance of individual PSMs (referred as spectral E -values) and the target-decoy approach to estimate false discovery rates (FDRs). See Gupta et al. [24] for the details of our probabilistic framework. Let P S be a peptide that generated S . A scoring function is adequate for S (with respect to a protein database ProteinDB ) if the correct peptide attains the maximal score in the database, that is, max P ε ProteinDB Score( P , S )=Score( P S , S ). A ‘good’ scoring function should satisfy the following three conditions. First, it should be adequate for the great majority of spectra. Second, the algorithm for PSM scoring should be fast. Third, the algorithm for computing statistical significance (for example, E -values) of PSMs should be fast and accurate. MS-GF+ uses a very simple dot-product scoring Score( P , S )= P *· S * after converting peptide P and spectrum S into peptide vector P * and spectral vector S * (the spectral vector was called the prefix-residue-mass spectrum in the previous publications [12] , [25] ). Conversion of a spectrum S into a spectral vector S * uses a probabilistic model that ensures that the resulting dot-product scoring is adequate [26] (first condition). At the same time, it makes scoring and computing accurate E -values fast [15] (second and third condition). This simple ‘dot-product’ scoring model contrasts with many other database search [2] , [4] , [27] , [28] and re-scoring [9] , [10] tools, using sophisticated scoring functions that often make it difficult to satisfy the third condition. MS-GF+ workflow MS-GF+ takes a spectral data set Spectra and a protein database ProteinDB as an input and outputs a set of scored PSMs along with E -value estimates. It uses open source application programming interfaces jmzML [29] , jmzReader [30] and jmzIdentML [31] , and supports the HUPO Proteomics Standard Initiative standard file formats—mzML [32] and mzIdentML [33] . Owing to these developments, MS-GF+ has been already adopted in many proteomics pipelines and post-processing tools. The workflow of MS-GF+ comprises the following four steps: generating spectral vectors, searching a protein database, computing E -values of PSMs and estimating FDRs. Below, we describe each step as well as how MS-GF+ takes advantage of high precision spectra. Generating spectral vectors A (non-modified) peptide is defined as a string over the alphabet A of 20 standard amino acids. Let A + be an extended amino acid set containing both unmodified and modified amino acids. For an (unmodified) amino acid a ε A , let Mod( a ) ⊂ A + be the set that contains a and all its modified amino acids. For example, if T (Thr) and T * (phosphorylated Thr) are in A + , Mod( T )={ T , T *}. Given a peptide P = a 1 … a k , define PV = pυ 1 … pυ k as a variant of P if pυ i ε Mod( a i ) for all i (1≤ i ≤ k ). MS-GF+ converts spectra into spectral vectors [12] , [25] . A spectral vector of a spectrum S is an M -dimensional vector with integer values, where M =PrecursorMass( S ) is the nominal precursor mass of S . Here we consider nominal precursor masses, representing that the sum of nominal masses of amino acids of the peptide generated the spectrum. As in many cases, the precise nominal precursor mass is unknown (for example, MS instruments often choose second or third isotope peak instead of mono-isotope peak from MS1 spectrum), multiple spectral vectors are generated separately for each possible nominal precursor mass and the score of a peptide of mass M is computed from the spectral vector of precursor mass M . The conversion from an experimental spectrum to a spectral vector proceeds as follows. A spectrum S ={( mz 1 , rank 1 ),…,( mz l , rank l )} is represented as a set of ranked peaks where the i th highest intensity peak gets rank i ( mz j and rank j represent m/z and rank of j th peak, respectively). An ion type is represented as a triplet of integers charge, offset and sign, where sign represents whether the ion type is a prefix ion (sign=1) or a suffix ion (sign=−1). For example, singly charged b-ions and y-ions correspond to ion types (1, 1, 1) and (1, 19, −1), respectively. Neutral losses and hydrogen transfers are also considered as ion types, for example, singly charged z·ions corresponds to (1, 3, −1). Given an ion type ion =( charge , offset , sign ), one can turn a spectrum S into S ion ={( mass 1 , rs 1 ),…, ( mass l , rs l )} using the following transformation: where [ x ] represents the closest integer to x and RankScore( ion , rank ) is a pre-computed function that takes an ion type ion and an integer rank, and returns a probabilistic log-likelihood score defined in refs 12 , 26 . It is noteworthy that 0.9995 is a rescaling constant for minimizing rounding errors (see Supplementary Table 1 ). In practice, RankScore( ion , rank ) also accounts for the location of the observed peak and the precursor charge and mass of the spectrum, which are omitted here for simplification. Ion types contributing to scoring are selected from the training set as described in Kim et al. [12] Assume that is a set of ion types that are selected. The spectral vector of S (denoted by S = ( s 1 ,…, s M )) is computed as follows: where RankScore( ion , ∞) represents the score given when ion is missing. We also define a peptide vector of a variant as follows. Let Mass( a ) be the nominal mass of a (possibly modified) amino acid a . For example, Mass( T )=101 and the mass of phosphorylated Thr is Mass( T *)=181. Given a variant PV = pυ 1 … pυ k , define the mass of PV as . Given a variant PV = pυ 1 … pυ k of mass M , we define its peptide vector (denoted by PV ) as a 0–1 vector ( m 1 ,…, m M ) with ( n −1) 1 s, such that m i =1 if i equals to Mass( pυ 1 )+…+Mass( pυ j )(1≤ j ≤ k ). The MS-GF+ score of a PSM ( PV , S ) is defined as if Mass( PV )=PrecursorMass( S ) and −∞ otherwise. The MS-GF+ score represents the log likelihood ratio described in ref. 26 . Searching a protein database We define ProteinDB + as the set of all variants (with respect to an extended amino acid set A + ) derived from ProteinDB . The goal of MS-GF+ database search is to solve the following problem: given a spectral data set Spectra and a protein database ProteinDB , for each spectrum S ε Spectra find a variant PV S , ProteinDB such that In contrast to a traditional spectrum-based MS/MS database search approach that compares each spectrum against all peptides, MS-GF+ uses an alternative peptide-based approach that computes the suffix array to compare each peptide against all spectra with the same precursor mass. See Supplementary Note 1 for the details of MS-GF+ approach to the database search. Computing E -values of PSMs The scores of PSMs reported by existing MS/MS database search tools are often poorly correlated with their E -values [34] . It is important to rank PSMs based on their E -values, because such ranking (rather than ranking based on ‘raw scores’) often dramatically increases the number of identified spectra under a given FDR [15] , [35] . Many database search tools estimate an E -value of a PSM based on an approximation of a tail of the score distribution specific to the spectrum using peptides in the database [27] , [28] . As this approach is known to result in biased estimates of E -values [15] , MS-GF+ adopted the generating function approach to rigorously compute E -values of PSMs using the score distribution of all peptides [15] . Our scoring model is essential here, because the generating function approach is easily applicable to the scoring functions that can be represented as a dot-product of vectors [24] . Adopting the generating function approach improves the accuracy of E -value estimates and increases the number of identified peptides as was recently confirmed by an independent work on applying it to the XCorr score in SEQUEST [35] . Given a spectrum S , a score threshold t , an extended set of amino acids A + and a database size N , we define E -value ( S , A + , t , N ) as the expected number of variants PV (as defined by A + ) with MSGFScore( PV , S )≥ t in a random protein database of size N . To compute E -value( S , A + , t , N ), we first compute spectral E-value E -value( S , A + , t ), the expected number of variants PV with MSGFScore( PV , S )≥ t given a single random peptide. A single random peptide models a random peptide starting at a fixed position in a random protein database. We consider a set of all possible (unmodified) peptides of length k (where k is a large number) and select a random peptide uniformly from this set (that is, the probability of selecting a peptide is ). In practice, to reflect different frequencies of amino acids in a database (for example, Leu is usually more common than Trp), we define the probability of a peptide P = a 1 … a k as , where Prob(a) is the frequency of amino acid a in a protein database. Note that this does not change the algorithm to compute the spectral E -values. We say that a peptide P produces a variant PV if PV is a variant of a prefix of P . For example, PEPT * and PEPTI are produced by PEPTIDE . Given a spectrum S , let V ( t ) be the set of all variants PV with MSGFScore( PV , S )≥ t . For every variant PV , there are 20 k −| PV | peptides of length k producing a variant PV (| PV | stands for the number of amino acids in PV ). Therefore, expected number of variants per random peptide with a score equal or better than t is As a variant is a string over the alphabet A + , this expression can be computed using the generating function approach [15] . Given a spectrum S with S = s 1 … s M , consider a directed acyclic graph called an amino acid graph G ( V , E , A + ) with V ={0, …, M } and E ={( i , j )| j − i ε Mass( a ) for a ε A + }, where the score of a vertex i is defined as s i , the probability of an edge is defined as , the score of a path is defined as the sum of scores of its vertices and the probability of a path is defined as the product of probabilities of its edges. A path in an amino acid graph represents a variant. Therefore, E -value( S , A + , t ) equals to the sum of probabilities of all paths from 0 to M with scores equal or better than t , and can be computed using parametric dynamic programming [15] , [26] , [36] . Although spectral E -values are useful for evaluating statistical significance of individual PSMs (independently of the database), they need to be transformed into E -value( S , A + , t , N ) to take into account the fact that the database search represents ‘multiple testing’ where multiple variants (arising from different database peptides) are scored against a spectrum [37] . E -values can be approximated as follows: where N is the size of the database. It is noteworthy that as protein databases contain many repeated peptides, it is important to reflect the effective size of the database that is estimated as the number of unique peptides of certain length. Estimating FDRs MS-GF+ estimates FDRs using the target decoy approach [38] , [39] . See Supplementary Note 2 for details. From low-precision to high-precision MS/MS spectra Mass spectrometers are usually divided into high-precision (denoted by H) and low-precision (denoted by L) instruments. Depending on whether the precursor and product ions are measured with low or high precision, the spectra are divided into LL, LH, HL and HH spectra (LH spectra are hardly ever used in proteomics studies). Although it may appear that extending the generating function approach from LL (as defined in ref. 15 ) to HL and HH spectra is a simple matter of tuning parameters that control the error tolerance, the situation is more complex. Here we explain how MS-GF+ takes advantage of high-precision product ion peaks. Let RMass( a ) be the real mass of an amino acid a . For a variant PV = pυ 1 … pυ k , let and RPrecursorMass( S ) be the real precursor mass of a spectrum S . We previously assumed that Mass( PV ) and PrecursorMass( S ) are integers and defined MSGFScore( PV , S )= PV · S if Mass( PV )=PrecursorMass( S ) and −∞ otherwise. It is noteworthy that this condition, although appropriate for LL spectra, is weak for HL and HH spectra, because it may be satisfied even when the real mass RMass( PV ) significantly deviates (for example, up to 0.5 Da) from RPrecursorMass( S ). Let represent the condition | a − b |<Δ. To take advantage of accurate precursor masses in HL and HH spectra, the condition Mass( PV )=PrecursorMass( S ) has to be redefined to , where Δ is the precursor mass tolerance. The database search problem with this modified definition of MSGFScore is now described by the following equation: where Spectra RMass( PV ) represents the set of spectra S ε Spectra satisfying . The key part of the generating function approach is the assumption that amino acids have integer masses (otherwise the parametric dynamic programming is difficult to implement). However, rounding amino acid masses to integers introduces errors. These rounding errors reduce after rescaling by 0.9995, making them appropriate for LL and HL spectra. However, for HH spectra the rounding errors remain too large even after rescaling, prohibiting MS-GF+ from benefiting from precise product ion peaks. A larger rescaling constant could better accommodate the mass accuracy, for example, the rescaling constant 274.335215 allows one to model spectra with 2.5 p.p.m. accuracy [40] . However, as the time complexity of the generating function algorithm is proportional to the rescaling constant, this rescaling makes computing E -values prohibitively slow. Here we present a new scoring algorithm taking advantage of the accurate product ion masses while not substantially increasing the running time of MS-GF+. In ref. 26 , we introduced an abstract model (seemingly unrelated to MS) that described a probabilistic process of transforming a Boolean string (peptide vector) into another Boolean string (spectral vector). This model, although adequate for low-precision spectra, needs to be modified for high-precision spectra. Here we model a peptide as a Boolean string (as before) but model a spectrum as a directed acyclic graph (DAG) and further apply a transformation of a Boolean string into a DAG for scoring real PSMs (see Methods for details). Our new idea behind the DAG modelling is as follows. Consider peaks at masses 100.01 and 157.4 that will be transformed into integer bins 100 and 157 in the Boolean string representation of the spectrum. After this transformation, we lose information about the exact difference between these two masses. However, in our new spectral DAG model this information is retained in edges of the spectral DAG and used in the scoring. Data sets Overall, we used 19 data sets (≈2.83 million spectra from human, yeast, mouse and Schizosaccharomyces pombe ) reflecting the diversity of MS data, corresponding to 17 distinct spectral types shown in Fig. 1 (see Methods for details on the data sets). For all these data sets, we benchmarked MS-GF+ against popular tools for peptide identification such as Mascot+Percolator. Comparison of MS-GF+ with Mascot+Percolator We compared the numbers of identified PSMs at 1% FDR for MS-GF+ and Mascot+Percolator (that is, PSMs reported by Mascot and re-scored by Percolator). Mascot+Percolator (Mascot version 2.3.02 integrating Percolator) was used for the comparison, because it represents a popular choice for peptide identification. We also tested several other tools such as SEQUEST, InsPecT [25] and OMSSA but do not report their results because they identified significantly fewer PSMs as compared with Mascot+Percolator. See Supplementary Table S2 for database search parameters. For all the 19 data sets, MS-GF+ identified significantly more PSMs compared with Mascot+Percolator ( Fig. 2 ). Figure 3a shows the benchmarking results for the five human data sets generated with varying fragmentations and instruments [20] . 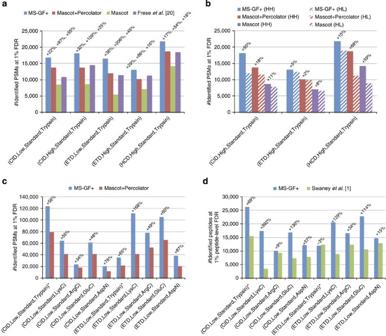Figure 3: Comparison of MS-GF+ and other tools for diverse spectral types. The numbers of identified PSMs (a–c) or peptides (d) at 1% FDR are shown. Numbers above bars represent the percentages of increase in the number of identifications for MS-GF+ compared with other tools. (a) Results for the human data sets with varying fragmentations and instruments. MS-GF+, Mascot+Percolator and Mascot results are shown along with the results in ref.20. Percolator greatly increased the number of identifications as compared with Mascot, but MS-GF+ outperformed Mascot+Percolator for all the data sets. (b) Increase in the number of identifications due to the availability of high-precision product ion peaks. For the three human data sets representing HH spectra, MS-GF+, Mascot+Percolator and Mascot were run using search parameters for HL spectra. The results of these searches (denoted by HL) are compared with the numbers of identifications for the regular searches (denoted by HH). HH searches identified more PSMs than HL searches for every tool and every data set. The difference was larger for CID and HCD than ETD spectra. (c) Results for the yeast data sets with varying fragmentations and enzymes. MS-GF+ and Mascot+Percolator results are shown. MS-GF+ outperformed Mascot+Percolator for all these data sets. (d) Comparison of MS-GF+ and the results in ref.1that used OMSSA along with in-house post-processing tools for the yeast data sets. The numbers of (unique) peptides at the peptide-level 1% are shown. In ref.1, only the number of identified peptides matched to proteins identified at 1% protein-level FDR was counted, while for MS-GF+ the number of identified peptides was counted regardless of their matched proteins. Percolator greatly increased the number of identifications as compared with Mascot, but for all these data sets MS-GF+ identified significantly more PSMs (17–38%) than Mascot+Percolator (see Supplementary Fig. S1 for Venn diagrams of MS-GF+ and Mascot+Percolator identifications). We also compared the number of identifications reported by the original study [20] , which also used Mascot+Percolator along with in-house pre- and post-processing tools. 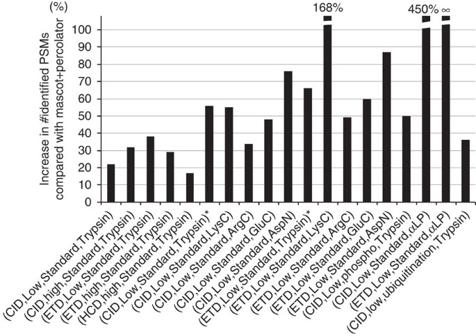In this comparison, MS-GF+ also showed an improved performance (identifying 16–55% more PSMs). Figure 2: Benchmarking MS-GF+ against Mascot+Percolator. Per cent increases in the number of identified PSMs for MS-GF+ compared with Mascot+Percolator for all 19 data sets. Each bar represents a spectral data set of a specified spectral type. For (CID, Low, Standard, Trypsin) and (ETD, Low, Standard, Trypsin), there are two corresponding data sets, one from human and the other from yeast. We distinguish them by adding ‘*’ to the yeast data sets. For the (CID, Low, Phosphorylation, Trypsin) and (CID, Low, Ubiquitination, Trypsin) data sets, the number of phosphorylated and ubiquitinated PSMs were counted instead of the number of all identified PSMs. For the (ETD, Low, Standard, αLP) data set, Mascot+Percolator identified no PSM. Figure 2: Benchmarking MS-GF+ against Mascot+Percolator. Per cent increases in the number of identified PSMs for MS-GF+ compared with Mascot+Percolator for all 19 data sets. Each bar represents a spectral data set of a specified spectral type. For (CID, Low, Standard, Trypsin) and (ETD, Low, Standard, Trypsin), there are two corresponding data sets, one from human and the other from yeast. We distinguish them by adding ‘*’ to the yeast data sets. For the (CID, Low, Phosphorylation, Trypsin) and (CID, Low, Ubiquitination, Trypsin) data sets, the number of phosphorylated and ubiquitinated PSMs were counted instead of the number of all identified PSMs. For the (ETD, Low, Standard, αLP) data set, Mascot+Percolator identified no PSM. Full size image Figure 3: Comparison of MS-GF+ and other tools for diverse spectral types. The numbers of identified PSMs ( a – c ) or peptides ( d ) at 1% FDR are shown. Numbers above bars represent the percentages of increase in the number of identifications for MS-GF+ compared with other tools. ( a ) Results for the human data sets with varying fragmentations and instruments. MS-GF+, Mascot+Percolator and Mascot results are shown along with the results in ref. 20 . Percolator greatly increased the number of identifications as compared with Mascot, but MS-GF+ outperformed Mascot+Percolator for all the data sets. ( b ) Increase in the number of identifications due to the availability of high-precision product ion peaks. For the three human data sets representing HH spectra, MS-GF+, Mascot+Percolator and Mascot were run using search parameters for HL spectra. The results of these searches (denoted by HL) are compared with the numbers of identifications for the regular searches (denoted by HH). HH searches identified more PSMs than HL searches for every tool and every data set. The difference was larger for CID and HCD than ETD spectra. ( c ) Results for the yeast data sets with varying fragmentations and enzymes. MS-GF+ and Mascot+Percolator results are shown. MS-GF+ outperformed Mascot+Percolator for all these data sets. ( d ) Comparison of MS-GF+ and the results in ref. 1 that used OMSSA along with in-house post-processing tools for the yeast data sets. The numbers of (unique) peptides at the peptide-level 1% are shown. In ref. 1 , only the number of identified peptides matched to proteins identified at 1% protein-level FDR was counted, while for MS-GF+ the number of identified peptides was counted regardless of their matched proteins. Full size image To figure out how each tool benefits from high-precision product ion peaks, for the three out of five human data sets representing HH spectra, we ran MS-GF+, Mascot+Percolator and Mascot using the parameters for HL spectra, that is, using 0.6 Da fragment mass tolerance for Mascot and Mascot+Percolator, and using the scoring model for low-precision spectra for MS-GF+. For every tool, the number of identifications was higher when the parameters for HH spectra were used, but the difference varied depending on the data set ( Fig. 3b ), and was negligible for ETD spectra. Figure 3c shows the comparison for the ten yeast data sets generated with varying fragmentations (CID or ETD) and enzymes (Trypsin, LysC, ArgC, GluC or AspN) [1] . Again, for all these data sets, MS-GF+ identified significantly more PSMs (34–168%) than Mascot+Percolator ( Fig. 3c ). In ref. 1 , using OMSSA (and in-house tools for pre- and post-processing), the authors reported the number of identified peptides at 1% peptide-level FDR that are matched to proteins identified at 1% protein-level FDR. We compared these numbers with the numbers of identified peptides at 1% peptide-level FDR using MS-GF+ ( Fig. 3d ). Note that this comparison is unfair because peptide identifications by MS-GF+ were not filtered out according to the protein that they are matched to. However, even after considering that, the results show that for most of the data sets MS-GF+ identified many more peptides than the original report. To see whether our scoring model can capture the fragmentation propensities specific to phosphopeptides, we generated a scoring parameter set for (CID, Low, Phosphorylation, Trypsin). For the mouse data set corresponding to (CID, Low, Phosphorylation, Trypsin), we compared the numbers of identified PSMs for MS-GF+ with and without using the phosphorylation-specific parameter set, Mascot+Percolator and InsPecT equipped with a dedicated scoring model for (CID, Low, Phosphorylation, Trypsin) [41] ( Supplementary Fig. S2a ). Interestingly, without phosphorylation-specific scoring parameters, MS-GF+ outperformed both tools, identifying 37% and 44% more PSMs than Mascot+Percolator and InsPecT, respectively. With phosphorylation-specific parameters, MS-GF+ identified 9% more PSMs (and 12% more PSMs of phosphopeptides), confirming that our scoring model successfully captures phosphorylation-specific fragmentation propensities. A similar result was obtained for a (CID, Low, Ubiquitination, Trypsin) data set ( Supplementary Fig. S3 ). We emphasize that MS-GF+ does not ‘know’ anything about the peculiarities of the phosphorylation or ubiquitination, and simply trains the scoring parameters in exactly the same way it does for other spectral types. This ability to easily train modification-specific scoring parameters for any modification will greatly benefit MS researchers studying PTMs. MS-GF+ for identifying peptides produced by a new protease αLP is a new protease with cleavage specificities somewhat ‘orthogonal’ to trypsin [23] . MS-GF+ was applied to the study of αLP using two S. pombe data sets corresponding to (CID, Low, Standard, αLP) and (ETD, Low, Standard, αLP). We ran Mascot+Percolator, OMSSA and MS-GF+ by specifying ‘None’ as an enzyme. As αLP produces peptides with different fragmentation propensities than tryptic peptides, Mascot+Percolator and OMSSA performed very poorly for this novel spectral type. In contrast, MS-GF+ identified 3,535 and 2,829 PSMs from the (CID, Low, Standard, αLP) and (ETD, Low, Standard, αLP) dataset using the scoring parameters for (CID, Low, Standard, Trypsin) and (ETD, Low, Standard, Trypsin), respectively ( Supplementary Fig. S2b ). The superior performance of MS-GF+ over Mascot+Percolator and OMSSA is because its scoring function is adequate for αLP peptides (correct peptide attains the maximal score) for a large portion of the spectra even when the search space is large (that is, no enzyme is specified). In fact, for the human data set corresponding to (ETD, Low, Standard, Trypsin), when no enzyme was specified and precursor mass tolerance 2.5 Da was used, MS-GF+ identified 10,937 PSMs, only 34% less as compared with the fully tryptic search with 7 p.p.m. precursor mass tolerance. Using the identified PSMs by MS-GF+, we trained scoring parameters for (CID, Low, Standard, αLP) and (ETD, Low, Standard, αLP). When these αLP-specific scoring parameters were used, the number of identified PSMs further increased to 4,788 (+35%) and 3,313 (+17%) for (CID, Low, Standard, αLP) and (ETD, Low, Standard, αLP), respectively, showing the usefulness of MS-GF+ for studies of new proteases. Thus, αLP represents a new alternative to trypsin, greatly increasing the PTM and protein sequence coverages, but generating spectra with unusual fragmentation propensities. We emphasize that the capabilities of αLP are not obvious when Mascot+Percolator or another tool is used, because it fails to identify αLP peptides. The details on αLP protease have been discussed in a separate paper [23] . Running time of MS-GF+ We measured the running time of MS-GF+ and Mascot+Percolator for LL, HL and HH spectra for various spectral types. For all the searches, MS-GF+ and Mascot+Percolator showed similar running times ( Supplementary Fig. S2c,d ). Our analysis and recent independent studies [35] , [42] , [43] , [44] showed that for diverse types of spectral data sets, MS-GF+ identifies more PSMs as compared with existing database search tools such as Mascot, X!Tandem, OMSSA, Crux, Comet and InsPecT, and statistical modelling tools such as Percolator. We emphasize that the generating function approach for accurately computing E -values significantly contributes to the improved performance of MS-GF+. For example, when E -values instead of MS-GF scores were used to cut off the results, the number of identified PSMs increased approximately by 70%, 50% and 20% for LL, HL and HH spectra, respectively. Although we focused on demonstrating MS-GF+ as a stand-alone tool, we emphasize that MS-GF+ can be combined with various other proteomics analysis tools. As we have decided to release MS-GF+ in 2012 well before this paper was prepared for a journal submission, MS-GF+ has already been integrated into the following pipelines and statistical modelling tools: Trans-Proteomics Pipeline [45] , Galaxy-P [46] , ProteoSuite [47] , IDPicker [11] , SearchGUI [48] , Scaffold [48] , ProteoSAFe, Skyline [49] and Percolator [10] , [50] . Peptide identification tools that combine the results of multiple database search tools such as MSblender [51] , Peptide-Shaker [52] and PepArML [53] also currently support MS-GF+. MS-GF+ is freely available at http://proteomics.ucsd.edu . Spectral DAG model Given an extended alphabet A + , we first explain how to convert a spectrum S into a labelled DAG G . G =( V , E ) has a vertex set V ={0, …, M =PrecursorMass( S )} and an edge set E ={( i , j )| j − i ε Mass( a ) for a ε A + }. For simplicity, suppose that the set of ion types ={(1, 0, 1)} (that is, only singly charged prefix ions with an offset zero contribute to the scoring). Given a constant δ called a fragment mass tolerance, two peaks of S with m/z x and y form a duo if y − x is approximately equal to a mass of an amino acid, that is, for a ε A + . The vertex label s i and the edge label s i,j of G are defined as follows: s i =1 if there exists a peak of mass x satisfying [0.9995· x ]= i and s i =0 otherwise; s i , j =1, if there exists a duo of peaks with masses x and y such that [0.9995· x ]= i and [0.9995· y ]= j , and s i , j =0 otherwise (see Fig. 4 for an example). 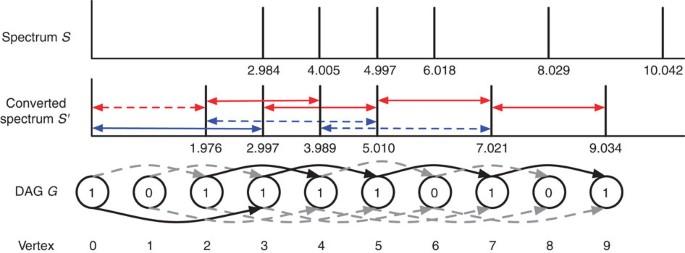Figure 4: Constructing a DAG in the case of two ‘amino acids’ with real masses 2.012 and 2.996. Assume that only singly charged b-ion with a real offset 1.008 contributes to the scoring. The spectrumSis converted intoS′ by shifting each peak by 1.008 to the left. Each arrowed line inS′ represents a pair of peaks separated approximately by 2 Da (blue) or 3 Da (red) that form a duo (solid) or does not form a duo (dashed) for a fragment mass tolerance 0.01 Da. A DAGGis constructed fromS′. The number in the vertex represents its label. The colour of the edge represents its label (0 for dashed grey and 1 for solid black). Figure 4: Constructing a DAG in the case of two ‘amino acids’ with real masses 2.012 and 2.996. Assume that only singly charged b-ion with a real offset 1.008 contributes to the scoring. The spectrum S is converted into S ′ by shifting each peak by 1.008 to the left. Each arrowed line in S ′ represents a pair of peaks separated approximately by 2 Da (blue) or 3 Da (red) that form a duo (solid) or does not form a duo (dashed) for a fragment mass tolerance 0.01 Da. A DAG G is constructed from S ′. The number in the vertex represents its label. The colour of the edge represents its label (0 for dashed grey and 1 for solid black). Full size image Let P = p 1 … p M be a Boolean string representing a peptide. Similar to the studies by Kim et al. [26] where a peptide string generates a spectrum string, we now assume that a peptide string generates a DAG. The probability of a peptide P generating a DAG G is defined as follows: where Prob( x | y ) is a 2 × 2 matrix representing the probability of a peptide character y (0 or 1) generating a vertex label x and Prob( x | y , z ) is a 2 × 4 matrix representing the probability of a pair of peptide characters y and z generating an edge label x ( Table 1 ). In practice, β 1 ≈ β 2 ≈ β 3 (see Table 1b ). Table 1 Probability table for generating directed acyclic graphs Full size table When applying this model for scoring a peptide P and a DAG G , we consider a test comparing two hypotheses: one assuming G is generated by P and the other assuming G is generated by an ‘empty’ string consisting of all zeros (denoted by O ). The log-likelihood score of ( P , G ) (denoted Score( P , G )) is defined as follows (see Fig. 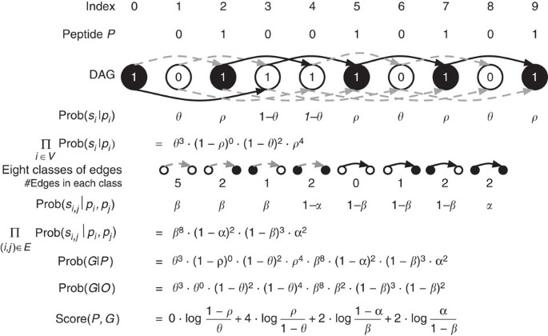Figure 5: Illustration of the MS-GF+ DAG scoring. The peptide ABAA is converted into its Boolean stringP=010010101 and the spectrumSis converted into a labelled DAGGas described in the text. The number in the vertex represents its label. The colour of the edge represents its label (0 for grey and 1 for black). The vertexiis coloured depending on the peptide characteri(white for 0 and black for 1). We also colour vertex 0 as black. The procedure to compute Score(P,G) is illustrated. All edges are partitioned into eight classes depending onsi,j,piandpj. For example, there are five edges withsi,j=pi=pj=0. 5 for an example): Figure 5: Illustration of the MS-GF+ DAG scoring. The peptide ABAA is converted into its Boolean string P =010010101 and the spectrum S is converted into a labelled DAG G as described in the text. The number in the vertex represents its label. The colour of the edge represents its label (0 for grey and 1 for black). The vertex i is coloured depending on the peptide character i (white for 0 and black for 1). We also colour vertex 0 as black. The procedure to compute Score( P , G ) is illustrated. All edges are partitioned into eight classes depending on s i,j , p i and p j . For example, there are five edges with s i,j = p i = p j =0. Full size image Note that the last equation assumes that only the edges ( i , j ) with p i = p j =1 contribute to the edge scoring because β 1 ≈ β 2 ≈ β 3 . In practice, we generate multiple DAGs for a single spectrum, one for each ion ε . To generate an ion DAG for ion=(charge, offset, sign) with a real offset r offset , (for example, real offset of the singly charged b-ion is 1.008), we first convert S ={( mz 1 , rank 1 ), …, ( mz l , rank l )} into S ′={( mass 1 , rank 1 ), …, ( mass l , rank l )} using the following transformation: Each peak of S representing ion corresponds to a peak of this converted spectrum S ′ representing an ion type (1, 0, 1). Therefore, the vertex and edge labels of the ion DAG for ion are defined as outlined before, but using S ′ instead of S ( Fig. 4 ). In reality, vertex and edge labels in the ion DAGs are integers rather than Boolean values. Given a converted spectrum S ′, we first remove all peaks ( x , rank ) if there exists another peak ( x ′, rank ′) where [0.9995· x ]=[0.9995· x ′] and rank > rank ′. The vertex label s i is defined as follows: s i = rank if there exists a peak ( x , rank ) satisfying [0.9995· x ]= i and s i =0 otherwise. For an integer m , let AminoAcid( m ) be the set of amino acids a ε A + satisfying Mass( a )= m (for example, AminoAcid(128)={Gln, Lys}). The edge label s i,j is defined as follows: s i,j =[100·min a εAminoAcid( j − i ) ( y − x −RMass( a ))] if there exists a duo of peaks with masses x and y such that [0.9995· x ]= i and [0.9995· y ]= j , and s i,j =∞ otherwise. The constant 100 is multiplied to discretize the real-valued errors into bins of size 0.01 Da. In this ion DAG representation, vertex labels encode the information on the intensities of individual peaks and the edge labels encode the information on the mass errors of pairs of peaks assuming they represent consecutive peaks of the same ion type. Note that edge labels take into account the spacing between peaks but do not take into account the peak intensities. Supplementary Note 3 describes how to integrate information from various ion DAGs into a single spectral DAG. Human data sets with varying fragmentations and instruments Five human data sets corresponding to the spectral types ( CID , Low , Standard, Trypsin), ( CID , High , Standard, Trypsin), ( ETD , Low , Standard, Trypsin), ( ETD , High ,Standard, Trypsin) and ( HCD , High , Standard, Trypsin) contain 38,401, 33,586, 30,451, 25,734 and 37,810 spectra, respectively. These data sets are generated in the Heck Laboratory (Utrecht University). HEK293 whole-cell lysates were digested by trypsin and analysed by LTQ-Orbitrap Velos (Thermo Fisher Scientific, Bremen), using combinations of one of the three fragmentation modes CID, ETD and HCD, and either ion trap or Orbitrap readout for product ion m/z . The detailed experimental procedures are described in ref. 20 . Yeast data sets with varying enzymes Ten yeast data sets corresponding to the spectral types ( CID , Low, Standard, Trypsin ), ( CID , Low, Standard, LysC ), ( CID , Low, Standard, ArgC ), ( CID , Low, Standard, GluC ), ( CID , Low, Standard, AspN ), ( ETD , Low, Standard, Trypsin ), ( ETD , Low, Standard, LysC ), ( ETD , Low, Standard, ArgC ), ( ETD , Low, Standard, GluC ) and ( ETD , Low, Standard, AspN ) contain 333,203, 278,336, 114,351, 81,669, 251,974, 72,463, 246,428, 204,860, 88,403 and 262,635 spectra, respectively. These data sets were generated in the Coon Laboratory (University of Wisconsin Madison). Yeast whole-cell lysates were digested separately, with either trypsin, LysC, ArgC, GluC or AspN, separated into 12 fractions via strong cation exchange chromatography and analysed in triplicate with an ETD-enabled LTQ-Orbitrap mass spectrometer, where peptide fragmentation was accomplished either with CID or ETD using the decision-tree acquisition mode [54] . We downloaded 180 (5 enzymes × 12 fractions × 3 replicates) spectrum files (Thermo RAW format) and converted each raw file into two mgf files, one containing CID and the other containing ETD spectra using ‘msconvert’ in ProteoWizard [55] with ‘no filtering’ option. The conversion was unsuccessful for 6 out of 180 files (5 from Arg-C and 1 from Glu-C digests). These six files were removed in the further analyses. The detailed experimental procedures are described in ref. 1 . Mouse data set of phosphopeptides A mouse data set corresponding to the spectral type (CID, Low, Phosphorylation , Trypsin) contains 181,093 spectra. This data set was generated from the Gygi Laboratory (Harvard Medical School). Nine mouse organ proteins were digested with trypsin and the resulting peptides were fractionated via strong cation exchange. Phosphopeptides were enriched via immobilized metal affinity chromatography and analysed in duplicates via LC-MS/MS on an LTQ-Orbitrap mass spectrometer. Out of nine organ tissues analysed, we used the spectra generated from the brain tissue. The detailed experimental procedures are described in ref. 21 . S. Pombe data sets with αLP digest Two data sets corresponding to the spectral type ( CID , Low, Standard, α LP ) and ( ETD , Low, Standard, α LP ) contain 49,167 spectra each. These data sets were generated in the Komives Laboratory (University of California, San Diego). The detailed experimental procedures to generate these data sets are as follows. Wild-type S. pombe cells were lysed in 50 mM Tris–HCl pH 8.0, 150 mM NaCl, 5 mM EDTA, 10% glycerol, 50 mM NaF, 0.1 mM Na3VO4, 0.2% NP40 and stored at −80 °C. The debris was pelleted and then the supernatant was collected. The pellet was extracted according to ref. 56 . Briefly, the pellet was resuspended in 200 μl of 0.1 M NaOH, 0.05 M ETDA, 2% SDS and 2% β-mercaptoethanol and incubated at 90 °C for 10 min. Acetic acid was added to 0.1 M and vortexed, followed by an additional incubation at 90 °C for 10 min before clarification by centrifugation and methanol/chloroform extraction. The pellet was resuspended in 100 mM Tris containing 0.1% sodium deoxycholate with TCEP at 5 mM. Free thiols were capped with N-ethylmaleimide. Excess reagent was removed by ultrafiltration with amicon-4 10 kDa centrifugal devices. The protein was then quantified and exchanged into 6 M guanidine for digestion overnight by αLP. The digests were quenched by the addition of formic acid to 1%, followed by desalting by sep-pak (Waters, Milford, MA). Peptides were then fractionated with electrostatic repulsion-hydrophilic interaction chromatography [57] . Fractions were assayed for protein concentration using a BCA assay and pooled into 18 fractions of equal protein concentration, evaporated to dryness and resuspended in 100 μl of 0.2% formic acid. Nano LC-MS/MS was performed with a LTQ XL mass spectrometer equipped with ETD. Ten microlitres of each fraction (≈1 μg) was injected onto a 12 cm × 75 μm I.D.C18 column prepared in house and eluted in 0.2% FA with a gradient of 5 to 40% Acetonitrile over 60 min followed by wash and re-equilibration totalling 90 min of MS data per run. The flow was split about 1:500 to a flow rate of about 250 nl min −1 . A survey scan was followed by data-dependent fragmentation of the four most abundant ions with both CID and ETD, with supplemental activation. The maximum MS/MS ion accumulation time was set to 100 ms. Fragmented precursors were dynamically excluded for 45 s with one repeat allowed. Training scoring parameters At the beginning of this study, we had five scoring parameter sets used in ref. 12 for the following five spectral types: (CID, Low, Standard, Trypsin), (CID, Low, Standard, LysN), (ETD, Low, Standard, Trypsin), (ETD, Low, Standard, LysN) and (ETD, Low, Standard, LysC). For this study, we constructed 20 new parameter sets using these 5 parameter sets as a starting point, using a newly developed programme called ScoringParamGen within the MS-GF+ package. To train scoring parameters for a new spectral type, MS-GF+ was run with an existing parameter set to identify PSMs at 1% FDR threshold, and using the identified PSMs as a training set a new parameter set was constructed. Supplementary Fig. S4 shows the scoring parameter sets contained in MS-GF+ and how they were constructed. We also tried to construct another generation of parameter sets using the existing parameter sets for the same spectral types, but this ‘iterative training’ hardly changed the number of identified PSMs. For some data sets, the same data set was used for both training and testing of the performance, raising concerns about overfitting. However, as shown in ref. 12 , MS-GF+ scoring parameter set characterizes a particular spectral type and is rather stable with respect to specific data sets. For example, for the human (CID, Low, Standard, Trypsin) data set, when the scoring parameter set trained from the same data set was used instead of the data set used in ref. 12 , the number of identified PSMs hardly changed. How to cite this article: Kim, S. and Pevzner, P. A. MS-GF+ makes progress towards a universal database search tool for proteomics. Nat. Commun. 5:5277 doi: 10.1038/ncomms6277 (2014).